A nanopore machine promotes the vectorial transport of DNA across membranes The transport of nucleic acids through membrane pores is a fundamental biological process that occurs in all living organisms. It occurs, for example, during the import of viral DNA into the host cell or during the nuclear pore complex-mediated transport of mRNA in and out the cell nucleus and has implications in nucleic acid drug delivery and gene therapy. Here we describe an engineered DNA transporter that is able to recognize and chaperone a specific DNA molecule across a biological membrane under a fixed transmembrane potential. The transported DNA strand is then released by a simple mechanism based on DNA strand displacement. This nanopore machine might be used to separate or concentrate nucleic acids or to transport genetic information across biological membranes. The use of natural components as building blocks in nanotechnology is advantageous because artificial biological devices are intrinsically able to interface with biological systems. However, adding new functions to proteins is not trivial because, despite important recent advances [1] , [2] , [3] , the folding of proteins cannot be easily predicted; moreover, to date the use of artificial protein systems in nanotechnology has been mainly limited to self-assembled protein arrays [4] , [5] . Recently, DNA has emerged as a preferred element to build and confer functionality to biologically based devices [6] . Self-assembled DNA nanostructures now range from compact 3D objects with a well-defined shape [7] , [8] , [9] to complex functional assemblies such as nanopores [10] , [11] that are capable of spanning artificial membranes [12] , [13] . The thermodynamics of DNA duplex formation have also been exploited to build systems that utilize strand hybridisation, branch migration, and dissociation for dynamic state reconfiguration [6] , [14] . Such DNA devices can switch configuration multiple times as detected by high and low FRET emission states [15] , act as computing elements for example to build molecular logic circuits that perform mathematical operations [16] or to reconfigure self-assembled DNA structures [17] and therefore have potential for imbedding control within molecular systems. Strand-displacement reactions have also been used to control mechanical actuation, as shown for DNA ‘walkers’ that can move along DNA tracks after the external addition of DNA reagents [18] , [19] , [20] , [21] , [22] , [23] , [24] . In the present work, we incorporate a DNA unit on the top of a protein nanopore to form a membrane-bound molecular machine that transports selected DNA molecules through the nanopore. The transported DNA is released by a strand-displacement reaction. Similarly to biological transporters, our device is capable of carrying a specific substrate across a biological membrane. dsDNA translocation through ClyA nanopores We used an engineered version of Cytolysin A (ClyA) from Salmonella typhi that was selected for its enhanced activity (ClyA-CS), solubility and favourable behaviour in planar lipid bilayers when compared with wild-type ClyA (ClyA-WT nanopores). In lipid bilayers, ClyA nanopores assembled with a preferred orientation ( Fig. 1a ) that could be easily assessed by the slightly asymmetrical current–voltage relationship of the pore [25] . The internal diameter of the ClyA dodecamer (3.3 nm at its narrower entrance [26] , Fig. 1a ) is larger than the diameter of dsDNA (2.2 nm for the B form), indicating that dsDNA should readily translocate through the pore when driven by an electrical potential. However, most likely because of the negatively charged residues lining the lumen of ClyA (the net lumen charge is −120), at physiological salt concentrations, DNA does not enter the nanopore [25] . Inspired by our previous work with alpha hemolysin (αHL) nanopores at high alkaline pH [27] , [28] , we tested the ability of DNA to translocate through ClyA-CS nanopores at high ionic strength, where the internal charges are screened. In 2.5 M NaCl, 15 mM Tris HCl, pH 7.5 and under +100 mV applied potential, the addition of 0.12 μM of biotinylated dsDNA 1 (290 bp, Supplementary Table S1 ) to the cis compartment produced transient current blockades ( I B ) to the open pore current ( I O ) showing a residual current ( I RES = I B / I O ) of 0.63±0.01 (mean±s.d., I B level 1* +100 =1.10±0.03 nA, mean±s.d., n =3 experiments), with a dwell time of 2.0±0.6 ms (mean±s.d.) because of the entry of the DNA into the lumen of the pore ( Fig. 1b ). The subsequent addition to the cis compartment of 0.3 μM of neutravidin, which forms a tight complex with biotin, converted the transient blockades into long-lasting current blockades (level 1 +100 =1.19±0.01 nA, mean±s.d., n =4) with a higher residual current value ( I RES+100 =0.68±0.01, mean±s.d., n =4). The open pore current could be restored by reversal of the applied potential to −100 mV ( Fig. 1b ). These results suggest that at positive applied potentials, dsDNA added to the cis compartment is transported through the pore to the trans chamber and that neutravidin prevents the full translocation of DNA through ClyA nanopores by forming a cis protein:DNA complex where the DNA occupies the full length of the pore ( Fig. 1c ). Trans complexes could also be formed at −100 mV (level 1 −100 =1.02±0.03 nA, mean±s.d., I RES−100 =0.62±0.01, mean±s.d., n =4) when the threading of the dsDNA:neutravidin complex is initiated from the trans side ( Fig. 1d ). 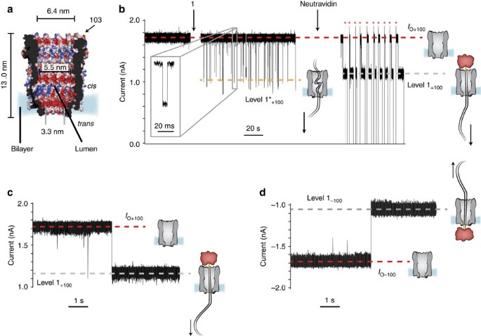Figure 1: dsDNA translocation through ClyA nanopores. On the right of the current traces, ClyA and neutravidin are depicted as grey and red cartoons, respectively, and the dsDNA is shown as a black double line. (a) A section through ClyA fromS. typhiconstructed by homology modelling from theE. coliClyA structure (PDB:2WCD, 90% sequence identity)25. ClyA is shown as surface representation and coloured according to the ‘in vacuo’ electrostatics (red for negative regions, and blue for positive regions, Pymol). The arrow shows one of the 12 residues of 103 (serine in the WT sequence). The pore dimensions are given considering the van der Waals radii of the atoms. (b) At +100 mV, the addition of 0.12 μM of 290 bp dsDNA1to thecisside of a ClyA nanopore provoked short current blockades ofIRES=0.63±0.01 (mean±s.d., levelIO+100=1.74±0.05 nA, mean±s.d. and level 1*+100=1.10±0.03 nA, mean±s.d.,n=3) that were because of the translocation of dsDNA through the pore. The addition of neutravidin to thecischamber converted the short current blockades to higher conductance and long-lasting current blockades withIRES+100=0.68±0.01 (mean±s.d., level 1+100=1.19±0.01 nA, mean±s.d.,n=4) due to the threading of DNA through the pore. The open pore current was restored by reversing the potential to −100 mV (red asterisks) and the stepping back to +100 mV. The inset shows a typical transient current blockade. (c) Details of a current blockade because of the formation of acispseudorotaxane at +100 mV. (d) Formation of atranspseudorotaxane at −100 mV by threading the dsDNA:neutravidin complex (see above) from thetransside (level 1−100=−1.02±0.03 nA, mean±s.d.,IRES-100=0.62±0.01, mean±s.d.,n=4). The electrical recordings were carried out in 2.5 M NaCl, 15 mM Tris HCl, pH 7.5 at 22 °C. Data were recorded by applying a 10-kHz low-pass Bessel filter and using a 20μs (50 kHz) sampling rate. Figure 1: dsDNA translocation through ClyA nanopores. On the right of the current traces, ClyA and neutravidin are depicted as grey and red cartoons, respectively, and the dsDNA is shown as a black double line. ( a ) A section through ClyA from S. typhi constructed by homology modelling from the E. coli ClyA structure (PDB: 2WCD , 90% sequence identity) [25] . ClyA is shown as surface representation and coloured according to the ‘in vacuo’ electrostatics (red for negative regions, and blue for positive regions, Pymol). The arrow shows one of the 12 residues of 103 (serine in the WT sequence). The pore dimensions are given considering the van der Waals radii of the atoms. ( b ) At +100 mV, the addition of 0.12 μM of 290 bp dsDNA 1 to the cis side of a ClyA nanopore provoked short current blockades of I RES =0.63±0.01 (mean±s.d., level I O+100 =1.74±0.05 nA, mean±s.d. and level 1* +100 =1.10±0.03 nA, mean±s.d., n =3) that were because of the translocation of dsDNA through the pore. The addition of neutravidin to the cis chamber converted the short current blockades to higher conductance and long-lasting current blockades with I RES+100 =0.68±0.01 (mean±s.d., level 1 +100 =1.19±0.01 nA, mean±s.d., n =4) due to the threading of DNA through the pore. The open pore current was restored by reversing the potential to −100 mV (red asterisks) and the stepping back to +100 mV. The inset shows a typical transient current blockade. ( c ) Details of a current blockade because of the formation of a cis pseudorotaxane at +100 mV. ( d ) Formation of a trans pseudorotaxane at −100 mV by threading the dsDNA:neutravidin complex (see above) from the trans side (level 1 −100 =−1.02±0.03 nA, mean±s.d., I RES-100 =0.62±0.01, mean±s.d., n =4). The electrical recordings were carried out in 2.5 M NaCl, 15 mM Tris HCl, pH 7.5 at 22 °C. Data were recorded by applying a 10-kHz low-pass Bessel filter and using a 20μs (50 kHz) sampling rate. Full size image Formation of a nanopore:DNA rotaxane To prove that dsDNA translocates through ClyA nanopores, we sought to build a DNA:nanopore rotaxane, in which a dsDNA molecule added to the trans side of a ClyA nanopore hybridizes with a second DNA strand on the cis side after threading through the lumen. Rotaxanes are supramolecular interlocked systems in which a linear unit (thread) passes through a macrocyclic ring and is tapped by two bulky substituents (stoppers) at each end. Such mechanically joined molecules have applications, for example, as switches in molecular electronics [29] or as components in molecular machines [30] . Rotaxanes have been made non-covalently from a variety of molecules including dsDNA [31] or by locking biotinylated ssDNA molecules threaded through an αHL nanopore with streptavidin on one side and a DNA hairpin on the other side (dsDNA cannot translocate through αHL) [32] . Here we used a ClyA nanopore, ClyA- 2, that contained 12 ssDNA molecules 2 (51 bases, Supplementary Table S1 , Fig. 2a ) covalently attached at their 5′-ends to cysteine residues introduced at the cis entrance of the pore (at position 103, Fig. 1a ) via disulphide linkages. 2 was designed to act as a rotaxane stopper. The thread 3 was a dsDNA molecule (59 bp, Fig. 2a and Supplementary Table S1 ) with an additional 31 nucleotides of ssDNA at the 5′-end that was designed to hybridize indirectly with the stopper at the cis side. 3 also contained a 3′-biotinylated linker that was used for complexation with neutravidin at the trans side. The linkage between the thread and stopper on the cis side was mediated by a bridging ssDNA molecule 4 ( Supplementary Table S1 , Fig. 2a ) that was complementary to the last 16 nucleobases of 2 and to the first 25 nucleobases of 3. Each time 3 and 4 were added to the trans compartment, at −100 mV the DNA thread was captured by the pore and not released upon reversal of the potential to +100 mV (level 2 +100 , I RES+100 =0.77±0.04, mean±s.d., n =4, Fig. 2b ), indicating that a DNA rotaxane was formed ( Fig. 2b ). Interestingly, at +100 mV the residual current of the rotaxane ( I RES+100 =0.77±0.04, mean±s.d.) was higher than the I RES values of the cis or trans protein:DNA complexes (pseudorotaxane) threads (0.68±0.01, mean±s.d., and 0.62±0.01, mean±s.d., respectively), suggesting that an unhybridized ssDNA stretch of 2 spanned the pore at positive potentials ( Fig. 2b ). The rotaxane could be disassembled by the addition of 20 mM dithiothreitol (DTT) to the cis chamber, which reduced the disulphide bond between 2 and ClyA and restored the open pore current at +100 mV ( Fig. 2c–e ). 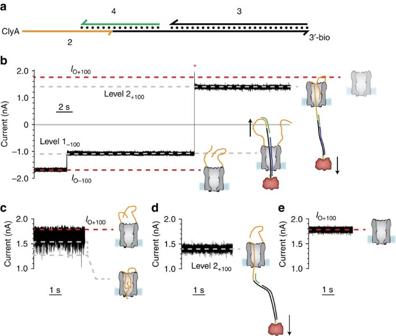Figure 2: Formation of a nanopore–DNA rotaxane. (a) Representation of the hybridization of the DNA molecules used to form the rotaxane. Arrowheads mark the 3′-ends of strands. The suffix bio indicates a biotin moiety. (b) Rotaxane formation. At −100 mV following the addition of the DNA hybrid3(1.0 μM) complexed with neutravidin (0.3 μM, tetramer) and oligo4(1.0 μM) to thetranscompartment, the open pore current of ClyA-2(IO−100=−1.71±0.07 nA, mean±s.d.,n=4) was reduced to level 1−100=−1.1±0.04 nA (mean±s.d.,IRES−100value of 0.64±0.02, mean±s.d.,n=4), indicating that dsDNA threaded the pore from thetransside. Stepping to +100 mV (red asterisk) produced a current block withIRES+100=0.77±0.04 (mean±s.d., level 2+100=1.31±0.09 nA, mean±s.d.,n=4), indicating that the DNA was still occupying the pore at positive applied potentials. Level 2 most likely corresponded to ssDNA2occupying the vestibule of the pore. Successive switching to positive and negative applied potentials did not restore the open pore current, confirming that a rotaxane was permanently formed. (c–e) Rotaxane removal. (c) At +100 mV, the ionic current through ClyA-2nanopores showed a multitude of fast current blockades (see alsoSupplementary Fig. S1), suggesting that the ssDNA molecules attached to thecisentrance transiently entered the lumen of the pore. (d) After the rotaxane was formed (Fig. 2b), at +100 mV the nanopore showed a steady ionic current (level 2+100), suggesting that a single DNA molecule was occupying the pore. (e) Twenty minutes after the addition of 20 mM DTT to theciscompartment, the DNA molecules atop the ClyA pore were removed by disulphide bond exchange and the open pore current at +100 mV was restored (IO+100=1.78±0.07 nA, mean±s.d.,n=4). The electrical recordings were carried out in 2.5 M NaCl, 15 mM Tris HCl, pH 7.5, at 22 °C. Data were recorded by applying a 10-kHz low-pass Bessel filter and using a 20 μs (50 kHz) sampling rate. Figure 2: Formation of a nanopore–DNA rotaxane. ( a ) Representation of the hybridization of the DNA molecules used to form the rotaxane. Arrowheads mark the 3′-ends of strands. The suffix bio indicates a biotin moiety. ( b ) Rotaxane formation. At −100 mV following the addition of the DNA hybrid 3 (1.0 μM) complexed with neutravidin (0.3 μM, tetramer) and oligo 4 (1.0 μM) to the trans compartment, the open pore current of ClyA- 2 ( I O−100 =−1.71±0.07 nA, mean±s.d., n =4) was reduced to level 1 −100 =−1.1±0.04 nA (mean±s.d., I RES−100 value of 0.64±0.02, mean±s.d., n =4), indicating that dsDNA threaded the pore from the trans side. Stepping to +100 mV (red asterisk) produced a current block with I RES+100 =0.77±0.04 (mean±s.d., level 2 +100 =1.31±0.09 nA, mean±s.d., n =4), indicating that the DNA was still occupying the pore at positive applied potentials. Level 2 most likely corresponded to ssDNA 2 occupying the vestibule of the pore. Successive switching to positive and negative applied potentials did not restore the open pore current, confirming that a rotaxane was permanently formed. ( c – e ) Rotaxane removal. ( c ) At +100 mV, the ionic current through ClyA- 2 nanopores showed a multitude of fast current blockades (see also Supplementary Fig. S1 ), suggesting that the ssDNA molecules attached to the cis entrance transiently entered the lumen of the pore. ( d ) After the rotaxane was formed ( Fig. 2b ), at +100 mV the nanopore showed a steady ionic current (level 2 +100 ), suggesting that a single DNA molecule was occupying the pore. ( e ) Twenty minutes after the addition of 20 mM DTT to the cis compartment, the DNA molecules atop the ClyA pore were removed by disulphide bond exchange and the open pore current at +100 mV was restored ( I O+100 =1.78±0.07 nA, mean±s.d., n =4). The electrical recordings were carried out in 2.5 M NaCl, 15 mM Tris HCl, pH 7.5, at 22 °C. Data were recorded by applying a 10-kHz low-pass Bessel filter and using a 20 μs (50 kHz) sampling rate. Full size image ssDNA and dsDNA blockades of ClyA-CS At high-positive applied potentials, the ionic current of ClyA- 2 nanopores fluctuated between the open pore level and several blocked pore levels ( Fig. 2c , Supplementary Figs S1 and S2a ), suggesting that the ssDNA molecules tethered to the top of the pore entered the lumen of ClyA but did not permanently thread to the trans side. Further supporting this interpretation, at +100 mV, the addition of a 90mer ssDNA with irrelevant sequence 5a ( Supplementary Table S1 ) complexed with neutravidin to the cis side of ClyA-CS provoked transient current blockades ( Fig. 3 ), which were converted into long-lasting DNA threading events upon the subsequent addition to the cis compartment of equimolar concentrations of the complementary ssDNA 5b ( Supplementary Table S1 , Fig. 3 ). To further investigate the capability of ssDNA to span the pore, we tested the ability of the DNA hybrid 3, which is formed by a 3′-biotinylated dsDNA section of 59 nucleobase pairs preceded by a 31-nucleotide 5′-overhang, to translocate through ClyA-CS pores. At +100 mV, the addition of 3 in complex with neutravidin to the cis side of a ClyA-CS pore provoked long-lasting current blockades with I RES+100 =0.69±0.01 (mean±s.d., Supplementary Fig. S6 ), the same I RES+100 value as observed for a cis pseudorotaxane (0.68, see above), suggesting that at this potential the DNA hybrid threads through ClyA and dsDNA spans the lumen of the pore. As the translocation of 3 can only be initiated from the ssDNA section of the DNA duplex, these results suggest that at +100 mV the ssDNA leading sequence of 3 is capable of translocating the lumen of ClyA. Interestingly, at +50 and +70 mV the current blockades were mostly transient ( Supplementary Fig. S6 ), suggesting that at this voltages ssDNA might not pass through the ClyA pore. The addition of strand 6 , which is complementary to the first 12 nucleobases of 3, also produced transient current blockades at +50 mV but the current blockades were permanent at +70 mV ( Supplementary Fig. S6 ), indicating that the additional dsDNA segment facilitated DNA translocation. 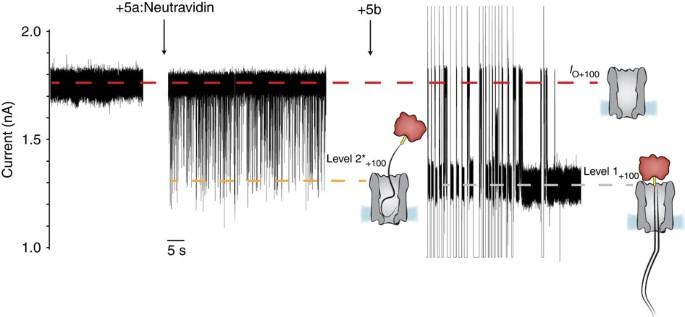Figure 3: ssDNA and dsDNA blockades of ClyA-CS. At +100 mV, the addition of 2.0 μM of a biotinylated ssDNA (5a) to thecisside of ClyA-CS nanopores in the presence of 0.6 μM neutravidin (tetramer) provoked transient current blockades (level 2*+100=1.24±0.02 nA, mean±s.d.,IRES+100=0.69±0.04, mean±s.d.,n=3), indicating that ssDNA entered the lumen of the pore but only transiently. The subsequent addition of 2.0 μM of the complementary ssDNA strand (5b) to theciscompartment converted the current blockades into permanent level 1+100blocks (1.22±0.13 nA, mean±s.d.,IRES+100=0.67±0.01, mean±s.d.,n=3), indicating that the dsDNA so formed spanned the entire length of the pore. After each DNA capture, the open pore was regenerated by manual reversal of the potential to −100 mV. Spikes above and below the open pore current level represent capacitive transients. The electrical recordings were carried out in 2.5 M NaCl, 15 mM Tris HCl, pH 7.5, at 22 °C. Data were recorded by applying a 10-kHz low-pass Bessel filter and using a 20μs (50 kHz) sampling rate. Figure 3: ssDNA and dsDNA blockades of ClyA-CS. At +100 mV, the addition of 2.0 μM of a biotinylated ssDNA ( 5a ) to the cis side of ClyA-CS nanopores in the presence of 0.6 μM neutravidin (tetramer) provoked transient current blockades (level 2* +100 =1.24±0.02 nA, mean±s.d., I RES+100 =0.69±0.04, mean±s.d., n =3), indicating that ssDNA entered the lumen of the pore but only transiently. The subsequent addition of 2.0 μM of the complementary ssDNA strand ( 5b ) to the cis compartment converted the current blockades into permanent level 1 +100 blocks (1.22±0.13 nA, mean±s.d., I RES+100 =0.67±0.01, mean±s.d., n =3), indicating that the dsDNA so formed spanned the entire length of the pore. After each DNA capture, the open pore was regenerated by manual reversal of the potential to −100 mV. Spikes above and below the open pore current level represent capacitive transients. The electrical recordings were carried out in 2.5 M NaCl, 15 mM Tris HCl, pH 7.5, at 22 °C. Data were recorded by applying a 10-kHz low-pass Bessel filter and using a 20μs (50 kHz) sampling rate. Full size image The threading of ssDNA or dsDNA into biological nanopores is often observed above a threshold potential [33] , [34] , [35] , [36] , [37] , [38] ( Supplementary Fig. S3 ) that can be tuned by altering the charge distribution of the lumen of the pore or by changing the ionic strength of the solution [27] , [39] . Therefore, our findings indicate that ssDNA has a higher threshold for threading through the pore than dsDNA. In solution, a generic ssDNA sequence has a relatively flexible (the persistence length of poly (dT) 40 is ~ 1.5 nm in 1 M KCl [40] ) but compact structure, which is formed by intrastrand base pairing and base-pair stacking interactions [41] , [42] , [43] , that needs to be disrupted to allow the entry of the ssDNA into the pore. By contrast, in dsDNA, intermolecular base pairing mediates duplex formation and short (<150 bp) dsDNA molecules behave as rigid rods (the persistence length of dsDNA in 1 M NaCl is ~ 50 nm (ref. 44 )) that do not need unfolding to thread through the ClyA pore. Therefore, the higher threshold for ssDNA threading through ClyA is most likely the result of a large entropic barrier because of the confinement of a flexible ssDNA molecule within the pore and to the uncoiling of the polymer before entering the nanopore. Sequence-specific DNA transport through a nanopore machine As at the positive applied potentials ssDNA threads the ClyA pore only transiently, ssDNA molecules attached to the cis entrance of ClyA will probe the cis solution. On the other hand, as at the positive applied potentials dsDNA threads the ClyA pore, when the ssDNA molecule becomes double-stranded (for example, by strand hybridization) the dsDNA strand will translocate through the pore and sample the trans solution. Therefore, we designed a nanopore:DNA device, in which the hybridization of a specific ssDNA molecule to the cis side of the ClyA- 2 nanopore promoted the translocation of the DNA duplex through the pore. The DNA duplex was then disassembled by a strand-displacement reaction ( Fig. 4a ), which resulted in the transport of the DNA cargo across the bilayer and the return of 2 to the cis chamber by movement against the applied potential. Conveniently, we found that at both +50 and +100 mV, the addition of a generic dsDNA molecule or a non-specific ssDNA molecule to the cis side of ClyA- 2 did not produce current blockades ( Fig. 4b and Supplementary Figs S4 and S5 ), indicating that the tethered ssDNA molecules produced a steric and/or electrostatic impediment that prevented or drastically reduced the entry of free dsDNA and also non-specific ssDNA from solution. Therefore, without the complication of dsDNA transport from solution, the ssDNA covalently attached atop the nanopore conferred specificity to the system by promoting the transport of selected ssDNA molecules while creating a barrier for the translocation of non-specific DNAs. 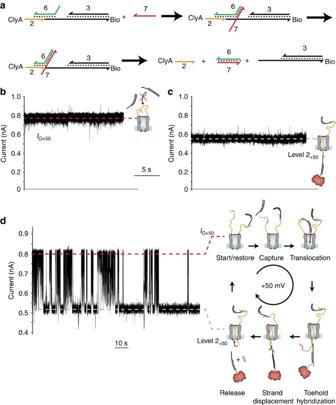Figure 4: Transport of DNA through ClyA nanopores. (a) Schematic representation of the strand-displacement reaction that promoted the release of DNA from the pore. The suffix bio indicates a biotin moiety. (b) At +50 mV and in the presence of3(0.3 μM), ClyA-2showed a steady open pore current (IO+50=0.85±0.01 nA, mean±s.d.,n=3), showing that the ssDNA strands attached to the pore did not thread through the lumen of the pore and prevented the translocation of dsDNA form solution. (c) The addition of the ssDNA strand6(40 nM) to thecischamber in the presence of the strand3and 0.3 μM neutravidin (tetramer) in thetranscompartment produced long-lasting current blockades withIRES+50=0.70±0.02 (mean±s.d., level 2+50=0.59±0.02 nA, mean±s.d.,n=5), indicating that the dsDNA hybrid threaded the pore. (d) The subsequent addition of 1 μM of7to thetranschamber (+50 mV) promoted the release of the DNA thread by a strand displacement reaction.2returned to theciscompartment against the applied potential and the open pore current was restored. Specific dsDNA molecules were then sequentially captured and released as shown by successive blocked and open pore currents. In this experiment, the applied potential was set to +50 mV and not to +100 mV as in the rest of this work. This is because at +100 mV ClyA-2occasionally produced long current blockades that were similar to typical events provoked by the capture of non-specific DNA (Supplementary Fig. S5c). Such current blockades were not observed at lower applied potentials; hence, we performed this experiment at +50 mV. In addition, at+50 mV the rate of DNA capture was lower than at +100 mV, and therefore the cycles of capture and release were more easily observed. The electrical recordings were carried out in 2.5 M NaCl, 15 mM Tris HCl, pH 7.5 at 22 °C. Data were recorded by applying a 2-kHz low-pass Bessel filter and using a 100μs (10 kHz) sampling rate. Figure 4: Transport of DNA through ClyA nanopores. ( a ) Schematic representation of the strand-displacement reaction that promoted the release of DNA from the pore. The suffix bio indicates a biotin moiety. ( b ) At +50 mV and in the presence of 3 (0.3 μM), ClyA- 2 showed a steady open pore current ( I O+50 =0.85±0.01 nA, mean±s.d., n =3), showing that the ssDNA strands attached to the pore did not thread through the lumen of the pore and prevented the translocation of dsDNA form solution. ( c ) The addition of the ssDNA strand 6 (40 nM) to the cis chamber in the presence of the strand 3 and 0.3 μM neutravidin (tetramer) in the trans compartment produced long-lasting current blockades with I RES+50 =0.70±0.02 (mean±s.d., level 2 +50 =0.59±0.02 nA, mean±s.d., n =5), indicating that the dsDNA hybrid threaded the pore. ( d ) The subsequent addition of 1 μM of 7 to the trans chamber (+50 mV) promoted the release of the DNA thread by a strand displacement reaction. 2 returned to the cis compartment against the applied potential and the open pore current was restored. Specific dsDNA molecules were then sequentially captured and released as shown by successive blocked and open pore currents. In this experiment, the applied potential was set to +50 mV and not to +100 mV as in the rest of this work. This is because at +100 mV ClyA- 2 occasionally produced long current blockades that were similar to typical events provoked by the capture of non-specific DNA ( Supplementary Fig. S5c ). Such current blockades were not observed at lower applied potentials; hence, we performed this experiment at +50 mV. In addition, at+50 mV the rate of DNA capture was lower than at +100 mV, and therefore the cycles of capture and release were more easily observed. The electrical recordings were carried out in 2.5 M NaCl, 15 mM Tris HCl, pH 7.5 at 22 °C. Data were recorded by applying a 2-kHz low-pass Bessel filter and using a 100μs (10 kHz) sampling rate. Full size image At +50 mV ( Fig. 4b ) or +100 mV (not shown), the addition of 3 to the cis side of ClyA- 2 did not produce current blockades, further confirming that the ssDNA molecules attached to ClyA- 2 prevent the entry of non-specific DNA in solution ( 3 cannot hybridize directly to 2 ). Nonetheless, after the addition to the cis chamber of 6 , which is complementary to the last 15 bases of 2 and to the first 12 nucleobases of 3 ( Supplementary Table S1 ), the dsDNA hybrid nanopore showed permanent current blockades with I RES+50 =0.70±0.02 (mean±s.d., level 2 +50 =0.59±0.02 nA, mean±s.d., n =5, Fig. 4c )—the hallmark of DNA capture. The translocation of 3 to the trans side was confirmed by the formation of a rotaxane upon addition of neutravidin (0.3 μM, tetramer) to the trans chamber ( Fig. 4c,d , Supplementary Fig. S3e–f ). Crucially, 6 was designed to include a 10-nucleotide 5′-single-stranded extension to serve as toehold for dissociation of the DNA thread ( Fig. 4a ). Gratifying, the addition to the trans chamber of 7 , a ssDNA molecule complementary to 6 ( Supplementary Table S1 ), released 3 from the nanopore by first hybridizing to the toehold and then promoting strand displacement ( Fig. 4a ). This was observed by the restoration of the open pore current because the ssDNA molecules tethered to ClyA returned to the cis side after 3 and 6 · 7 duplex were released from the pore ( Fig. 4d ). Remarkably, the nanopore showed several successions of open and blocked current levels, reflecting cycles of capture, translocation and release, as the DNA cargos were captured from the cis chamber, transported through the pore and released to the trans chamber ( Fig. 4d ). The restoring of the open pore current was not due to the spontaneous retraction of the dsDNA duplex to the cis compartment because at +50 mV dsDNA molecules could not exit the pore against the applied potential ( Supplementary Fig. S3d ). In addition, a previous study found that the binding to streptavidin of single biotinylated PEG molecules tethered to the cis side of a αHL pore has an on-rate of 3.8 × 10 6 M −1 s −1 (ref. 45 ), indicating that the DNA·neutravidin complex formed in about 200 ms, which is faster than the observed DNA release time (1.7±0.4 s, mean±s.d., n =4). Releasing kinetics and cycling Through the analysis of event lifetimes ( τ off ) of the blocked pore current (level 2), we measured a kinetic constant of 0.59±0.14 μM −1 s −1 for the strand-displacement reaction at the trans chamber. This value corresponded reasonably well with the ~ 1 μM −1 s −1 rate constants measured for equivalent strand-displacement reactions in ensemble experiments [46] , further confirming that the dsDNA segment of the DNA thread is largely exposed to the trans solution (that is, it is not confined within the pore lumen). We observed an average of 41±22 (mean±s.d., n =7) cycles before the DNA thread could no longer be released or captured. Occasionally, the cycling spontaneously started again after a few tens of minutes. As we observed more cycles while the bridging oligo 6 and release oligo 7 were high-performance liquid chromatography-purified, it is likely that the DNA strands contained contaminants of DNA molecules of defected synthesis (for example, with shorter toeholds or imperfect complementary sequences), which slowed down or stopped the strand-displacement reaction operated by 7 or failed to capture the DNA thread operated by 6 . Energy landscape of DNA transport At positive applied potential, the transport of DNA from the cis compartment to the trans compartment is energetically favourable because the DNA molecules diffuse down a concentration and an electrical potential gradient. However, the threading of ssDNA was not observed experimentally, revealing a large and mainly entropic energy barrier for ssDNA transport through the pore (see above). By contrast, the threading of tethered dsDNA was observed mainly because duplex hybridization atop of the pore reduced the entropic energy barrier for DNA translocation (see above). Once the tethered dsDNA was on the trans side of a ClyA- 2 pore, the cargo dsDNA would eventually be slowly and spontaneously released to the trans chamber. In this work, this process is catalysed by the strand-displacement reaction operated by the fuel strand in the trans chamber. Finally, the translocated tethered ssDNA 2 retracted against the applied potential to the cis compartment. Presumably, the return to the cis compartment against the potential and the formation of a compact ssDNA structure in the cis compartment was favoured over the confinement of a ssDNA strand in the pore under +50 mV and the formation of a smaller compact ssDNA structure in the trans compartment. In this work, we have built a membrane-imbedded DNA transporter that is able to selectively shuttle DNA molecules across a phospholipid membrane. Notably, this molecular machine does not allow the translocation of either ssDNA or non-tethered dsDNA; it works without external intervention (that is, at a constant transmembrane potential) and is modulated by two single-stranded DNA molecules: one attached to the pore that promotes the capture of DNA and the other in the trans solution that behaves as ‘fuel’ and promotes the release of a transported DNA cargo. Materials DNA was purchased from Integrated DNA Technologies (IDT). 6 and 7 were high-performance liquid chromatography-purified by the maker. Neutravidin was acquired from Thermo Fisher and 1,2-diphytanoyl- sn -glycero-3-phosphocholine from Avanti Polar Lipids. β-Dodecyl maltoside (DDM) was purchased from GLYCON Biochemicals GmbH. Enzymes were bought from Fermentas and all other materials from Sigma, unless otherwise specified. Protein preparation ClyA-CS contains five mutations relative to the ClyA-SS sequence: S87C, L99Q, E103G, F166Y and K294R. Monomers containing a C -terminal oligo-histidine tag were expressed in E. coli BL 21 cells and the soluble fraction purified using Ni-NTA affinity chromatography. ClyA dodecamers were formed by the addition of 0.2% DDM and were separated from monomers using blue native polyacrylamide gel electrophoresis. The lowest band of oligomeric ClyA-CS was extracted and stored at 4 °C. ClyA- 2 nanopores were prepared by covalently attaching 2 to a ClyA protein, in which the two WT cysteine residues (positions 87 and 285) were substituted with serine (ClyA-SS), and a cysteine was introduced at position 103 (aspartate in the WT gene; ClyA-SSC 103 ). ClyA-SSC 103 was constructed from ClyA-SS, which also encoded a Gly-Ser-Ser linker followed by a C -terminal hexahistidine tag by using the megaprimer method [47] using Phire Hot Start DNA Polymerase (Finnzymes). The DNA (5′-TTTTTTTTTATCTACGAATTCATCAGGGCTAAAGAGTGCAGAGTTACTTAG-3′), containing a protected thiol group attached to the 5′ hydroxyl of the DNA strand via a C6 linker (5ThioMC6-D, IDT), was then conjugated to ClyA-SSC 103 monomers, purified and oligomerized in DDM solutions [25] . Purified oligomers were stored at −80 °C in 20% glycerol. DNA preparation 1 was made using PCR amplification of a pT7-ClyA-WT DNA template using a 5′ biotinylated forward primer (bio-5′-TAATACGACTCACTATAGGG-3′) and a non-biotinylated reverse primer (5′-CATCAGCAGCACTTTGATATCGCCCACC-3′) using Taq DNA Polymerase from REDTaq ReadyMix PCR Reaction Mix (Sigma). After a maximum number of 35 cycles, the PCR products of 24 reaction tubes (50 μl each tube) were purified by using a PCR quick purification kit (QIAGEN), and the size of the construct was checked by using a 2% agarose gel (TAE buffer). The typical product concentration was ~ 200 ng μl −1 . 3 was formed by incubating a 3′-biotinylated ssDNA molecule (5′-GGATGACCTGATCCAGATATTTATTATACAGGTCCAGCGCACCGTCAGCCCAATCGCACTTTTC ACAAAAAGAGAGAGAGATCGATTACC-3′-bio, 3a ), with a 20% excess of a partially complementary ssDNA (5′-GGTAATCGATCTCTCTCTCTTTTTGTGAAAAGTGCGATTGGGCTGACGGTGCGCTGGAC-3′, 3b , Supplementary Table S1 ). The temperature was brought to 95 °C for 1 min and then decreased stepwise to room temperature. At around the estimated annealing temperature, the temperature was decreased in 2°C steps, each held for 1 min. The hybrid DNA was then purified from the excess of ssDNA with affinity chromatography using a biotin-binding column containing monomeric avidin immobilized on agarose beads (Thermo Scientific Pierce). 3 was eluted in Biotin Blocking/Elution Buffer according to the protocol and stored at −20 °C without further purification. Typically, a DNA concentration of ~ 400 ng μl −1 was obtained. The size of the dsDNA was checked by using a 2% agarose gel in TAE buffer. The purified dsDNA was stored at −20 °C in the presence of 1 mM EDTA. Electrical recordings and data analysis Artificial planar lipid bilayers were prepared as described [48] . If not otherwise specified, the signal was collected at a sampling rate of 50 kHz after processing with a 10-kHz Bessel filter. The lipid bilayer was formed by the addition of 1–2 μl of a 10% solution of 1,2-diphytanoyl-sn-glycero-3-phosphocholine in pentane. The electrical potential was applied by using Ag/AgCl electrodes submerged in agar bridges (3% w/v low melt agarose in 2.5 M NaCl buffer). The applied potential refers to the potential of the working electrode connected to the trans compartment of the apparatus. ClyA nanopore solutions (0.01–0.1 ng ml −1 ) were added to the cis compartment, which was connected to the ground electrode. After the insertion of a single pore, excess protein was removed by several cycles of perfusion. Electrical recordings were carried out in 2.5 M NaCl, 15 mM Tris HCl, pH 8.0, at 22 °C. The errors indicate the standard deviation from the average for at least three independent repeats, the number of which is indicated by ‘ n ’. The duration of the DNA release cycle was measured by fitting the dwell time of the blocked pore current (level 2 +50 ) to a single exponential (logarithmic binning, 10 bin per decade). I O and I B values were calculated from Gaussian fitting to all-point histograms of the open pore and blocked pore currents, respectively. How to cite this article: Franceschini, L. et al. A nanopore machine promotes the vectorial transport of DNA across membranes. Nat. Commun. 4:2415 doi: 10.1038/ncomms3415 (2013).